Brownian motion and quantum dynamics of magnetic monopoles in spin ice Spin ice illustrates many unusual magnetic properties, including zero point entropy, emergent monopoles and a quasi liquid–gas transition. To reveal the quantum spin dynamics that underpin these phenomena is an experimental challenge. Here we show how crucial information is contained in the frequency dependence of the magnetic susceptibility and in its high frequency or adiabatic limit. The typical response of Dy 2 Ti 2 O 7 spin ice indicates that monopole diffusion is Brownian but is underpinned by spin tunnelling and is influenced by collective monopole interactions. The adiabatic response reveals evidence of driven monopole plasma oscillations in weak applied field, and unconventional critical behaviour in strong applied field. Our results clarify the origin of the relatively high frequency response in spin ice. They disclose unexpected physics and establish adiabatic susceptibility as a revealing characteristic of exotic spin systems. In spin ice materials like Ho 2 Ti 2 O 7 or Dy 2 Ti 2 O 7 (refs 1 , 2 , 3 , 4 , 5 , 6 , 7 ) magnetic rare earth ions (for example, Ho, Dy) occupy a lattice of corner-linked tetrahedra. In the low temperature spin ice state two atomic magnetic moments or ‘spins’ point into, and two point out of each tetrahedron. This is equivalent to the ice rule that determines proton configurations in water ice [1] , [2] , and hence spin ice has a residual entropy equal to the Pauling entropy of water ice [3] . The thermodynamic properties of spin ice are well described by a classical spin Hamiltonian with a dominant dipole–dipole interaction [4] , [8] . The self-screening of the latter establishes the ice rule ground state [4] , but this property does not extend to excited states [5] . A spin flip out of the ice rule manifold creates a dipolar magnetic excitation that may fractionalize to produce free defects. These inhabit the diamond lattice formed by tetrahedron centres and behave as magnetic monopoles on account of the integrated dipole–dipole interaction [5] , [6] . The spin ices are part of the family of rare earth pyrochlores, a series of frustrated magnets for which collective quantum effects have been widely discussed [9] , [10] , [11] , [12] , [13] , [14] , [15] . Recent theoretical work [16] , [17] does not rule out the possibility that such effects may be relevant to Ho 2 Ti 2 O 7 and Dy 2 Ti 2 O 7 but, to a good approximation, the monopoles may be treated as classical objects, with local quantum mechanics setting local parameters such as attempt frequencies. The magnetic monopole current density in spin ice is defined as the rate of change of magnetization: J =∂ M /∂ t , with the conductivity proportional to the monopole density [6] . However, even in an infinite system, magnetic monopoles in spin ice cannot sustain a direct current (dc), on account of the destruction of the spin ice entropy by magnetization of the system [6] . This means that dc ‘magnetricity’ in spin ice [18] , [19] is necessarily transient [20] , [21] . Alternating current (ac) ‘magnetricity’ does not suffer from this limitation as monopoles can in principle be driven indefinitely back and forth by an oscillating magnetic field. The theory of ac-current [6] has not yet been tested as existing ac-magnetization studies either precede the theory [22] , [23] or focus on the low temperature regime [24] , [25] where complicating factors are expected [19] , [20] , [21] . Here, we present the first experimental test of the theory of Ryzhkin [6] , where we add experimental support to a number of ideas and arguments about monopole diffusion [20] , [21] , [26] and spin tunnelling [22] , [27] , [28] , and derive new information on the microscopic processes involved. Our dynamical magnetization measurements also estimate the isothermal susceptibility χ T and the adiabatic susceptibility χ S . Although the former is a much discussed magnetic response function, the latter is typically neglected. We also report a striking contrast between the temperature dependence of χ S and χ T in weak applied field, showing that χ T is best interpreted as a spin response, while χ S is best interpreted as a monopole response. This contrast has its root in the fact that configurational entropy ultimately confines the monopoles when they are driven by a magnetic field [6] . Finally, in strong applied field along the cubic [111] direction, spin ice exhibits a liquid–gas type phase transition with a critical point [29] at μ 0 H C =0.929 T, T C =0.36 K. This transition has been interpreted as a monopole condensation [5] and has been treated in renormalization group theory [30] . We extend our comparison of χ T and χ S to the ‘supercritical regime’ at T > T C , where we observe strong signatures of critical behaviour and find that monopoles behave increasingly like dipole pairs, in agreement with the comments of Shtyk and Feigel’man [30] . General features of the magnetic response in spin ice The temperature and field regimes probed in this paper are illustrated in Fig. 1 . In the figure we show the relationship between monopoles and dipoles in spin ice and we broadly define regimes of monopolar response and dipolar response. It should be emphasized that, as in other cases where novel quasiparticles accurately account for the low-energy physics, monopole and spin descriptions are never in conflict. Instead, certain properties are best discussed in terms of spins and others are best discussed in terms of monopoles. Our study clarifies how this division should be made. 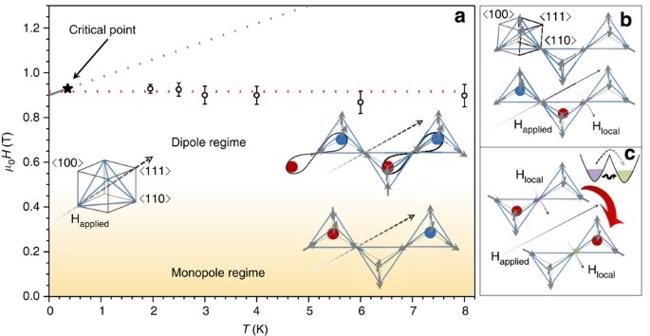Figure 1: Field-temperature phase diagram of spin ice. (a) Dy2Ti2O7with. The full line is a line of first order phase transitions, terminating in a classical critical point, that has been interpreted as a monopole condensation5. Monopoles are deconfined in zero field but become confined in an applied field. The right hand diagrams show how the monopoles reform flippable spins or dipole pairs near the critical field. Dotted lines are guides to the eye. Experimental points with error bars (s.d.) show the applied field of the maximum in the adiabatic susceptibility measured here.Hopping of emergent magnetic monopoles: fragment of spin ice’s cubic pyrochlore lattice, which consists of corner-linked tetrahedra, showing spin configurations (arrows). (b) Illustrates crystallographic axes, the applied field direction and how internal fields may be transverse to the local spin direction. Blue (red) circles represent negative (positive) monopoles. (c) Illustrates how a monopole hop can be associated with a spin flipped by a transverse field or a tunnelling event through a potential barrier. Figure 1: Field-temperature phase diagram of spin ice. ( a ) Dy 2 Ti 2 O 7 with . The full line is a line of first order phase transitions, terminating in a classical critical point, that has been interpreted as a monopole condensation [5] . Monopoles are deconfined in zero field but become confined in an applied field. The right hand diagrams show how the monopoles reform flippable spins or dipole pairs near the critical field. Dotted lines are guides to the eye. Experimental points with error bars (s.d.) show the applied field of the maximum in the adiabatic susceptibility measured here. Hopping of emergent magnetic monopoles : fragment of spin ice’s cubic pyrochlore lattice, which consists of corner-linked tetrahedra, showing spin configurations (arrows). ( b ) Illustrates crystallographic axes, the applied field direction and how internal fields may be transverse to the local spin direction. Blue (red) circles represent negative (positive) monopoles. ( c ) Illustrates how a monopole hop can be associated with a spin flipped by a transverse field or a tunnelling event through a potential barrier. Full size image One of our key results is that in spin ice, the adiabatic susceptibility χ S is finite, with the ratio χ S / χ T increasing with increasing applied static magnetic field. This basic observation is emphasized in Fig. 2 , which displays representative experimental data at T =1.95 K, in different applied static magnetic fields. The figure clearly shows the presence of a finite offset, χ S , in the limit of infinite frequency. 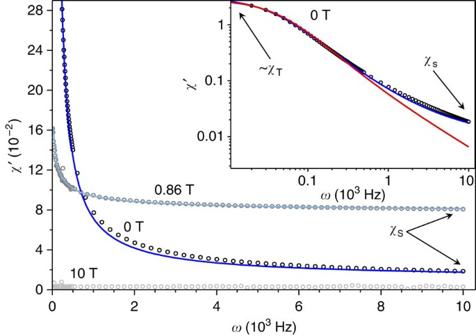Figure 2: Finite adiabatic susceptibility in spin ice. The adiabatic () and isothermal () susceptibilities are estimated as the real part of the frequency dependent susceptibilityin the limitsand, respectively, as indicated in the main plot. Experimental data are atat applied static magnetic field(black circles),(grey circles) and(light grey circles). At 10both susceptibilities are nearly zero. At 0.86, the two are of similar magnitude. At zero applied field, but still finite. The respective lines are the fit to a Cole–Cole model (see text). The inset shows thedata on log–log scales. The clear deviation from a linear curve at largeconfirms the presence of a finite offset,. Here the blue line is the fit to the Cole–Cole function using finiteand the red line is the same fit withconstrained to be zero. Figure 2: Finite adiabatic susceptibility in spin ice. The adiabatic ( ) and isothermal ( ) susceptibilities are estimated as the real part of the frequency dependent susceptibility in the limits and , respectively, as indicated in the main plot. Experimental data are at at applied static magnetic field (black circles), (grey circles) and (light grey circles). At 10 both susceptibilities are nearly zero. At 0.86 , the two are of similar magnitude. At zero applied field , but still finite. The respective lines are the fit to a Cole–Cole model (see text). The inset shows the data on log–log scales. The clear deviation from a linear curve at large confirms the presence of a finite offset, . Here the blue line is the fit to the Cole–Cole function using finite and the red line is the same fit with constrained to be zero. Full size image Magnetic relaxation in zero DC field The theory of Ryzhkin [6] applies the thermodynamics of irreversible processes to the problem of magnetic monopole transport in spin ice, specifically exploiting the spin ice-water ice analogy and the Jaccard theory of defect motion in water ice [31] . It is shown that the usual entropy gain of driving a current (in this case a monopole current) is opposed by the entropy loss in magnetization of the system. A current is only possible when the dynamical magnetization M ( t ) is less than its equilibrium value χ T H . The expression for the frequency dependent susceptibility of spin ice, χ (ω) calculated in Ryzhkin’s theory [6] therefore depends on both χ T and the monopole transport coefficients. This result is discussed at length in Ref. 32 where it is suggested, following the classical thermodynamic arguments of Casimir and Du-Pré [33] , that for practical purposes, the expression for the susceptibility calculated in Ryzhkin’s theory [6] should be modified to include a finite adiabatic susceptibility χ S . With this modification, the result of Ryzhkin’s theory [6] becomes: where τ is a relaxation time. Although this expression looks like that for ordinary paramagnetic relaxation, there is an important difference, in that τ is a function of monopole rather than spin parameters. It may be written τ −1 = μ 0 uQx / V 0 χ T where u is the monopole mobility, Q =4.266 × 10 −13 J T −1 m −1 the monopole charge [5] , x the total monopole density per diamond lattice site, and V 0 =1.29 × 10 −28 m 3 the volume per diamond lattice site [32] . The relaxation time τ therefore depends on three temperature-dependent parameters: u ( T ), x ( T ) and χ T ( T ). Of these, only the isothermal susceptibility χ T ( T ) can be directly measured. The density x ( T ) evolves with temperature in a way that cannot be expressed in closed form [26] , but we have estimated it with sufficient accuracy by fitting specific heat data to Debye–Hückel theory (refs 26 , 34 ), Methods and Supplementary Note 1 ). Knowledge of the experimental x ( T ) and χ T ( T ) allows us to determine the monopole mobility u ( T ) by dividing our measured τ −1 ( T ) by x ( T )/ χ T ( T ). In practice we found the assumption of a single relaxation time to be too restrictive, and therefore considered a modified model with one extra parameter introduced to describe a distribution of relaxation times. The Cole–Cole model [35] , which describes a roughly Gaussian distribution of log-relaxation times, was chosen because it was found to fit the experimental data and has some physical justification in that its approximately Gaussian cutoff at high frequency is consistent with a monopole hopping model: certain other commonly-used models are less suitable in this regard ( Supplementary Fig. S1 and Supplementary Note 2 , for a discussion). The expression used to fit the data therefore took the form: where α is the Cole–Cole parameter that determines the width of the log-relaxation time distribution (see Methods). Representative experimental data and results, along with characteristic fits, are shown in Fig. 3 . The model fits the experimental data well at T >3.5 K but describes only the high frequency part at the lowest temperatures (for details of fits in this range, Supplementary Fig. S1 ). 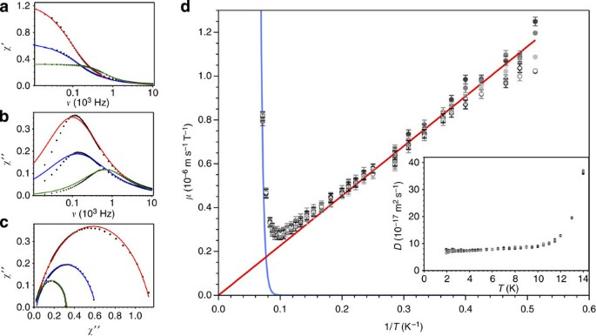Figure 3:Ac-magnetricity and monopole diffusion in spin ice,Dy2Ti2O7. A representative fit to the ac-magnetization data at: (a) real and (b) imaginary susceptibilities and (c) Cole–Cole plot (an argand diagram). The lines (red,T=4.5; blue, T=8; green, T=14) fit all data with the same set of four parameters at a given temperature:,,and, as defined in the text. (d) Monopole mobility measured at applied fields(full black circles), 3 (full dark grey), 10 (full light grey), 18.5 (open black) and 38.5 (open grey). Error bars represent the s.d. The red line iswhere. This is characteristic of Brownian diffusion of monopoles with a temperature-independent diffusion constant (inset). The blue line iswhere,, characteristic of a previously identified Orbach-like spin flip process arising from the coupling to excited crystal field states. This process is extinct below, giving way to monopole diffusion as the cause of magnetic relaxation in spin ice. Figure 3: Ac-magnetricity and monopole diffusion in spin ice, Dy 2 Ti 2 O 7 . A representative fit to the ac-magnetization data at : ( a ) real and ( b ) imaginary susceptibilities and ( c ) Cole–Cole plot (an argand diagram). The lines (red, T =4.5 ; blue, T=8 ; green, T=14 ) fit all data with the same set of four parameters at a given temperature: , , and , as defined in the text. ( d ) Monopole mobility measured at applied fields (full black circles), 3 (full dark grey), 10 (full light grey), 18.5 (open black) and 38.5 (open grey) . Error bars represent the s.d. The red line is where . This is characteristic of Brownian diffusion of monopoles with a temperature-independent diffusion constant (inset). The blue line is where , , characteristic of a previously identified Orbach-like spin flip process arising from the coupling to excited crystal field states. This process is extinct below , giving way to monopole diffusion as the cause of magnetic relaxation in spin ice. Full size image Figure 3d shows the temperature evolution of the monopole mobility, u ( T ). At T >10 K the apparent mobility diverges in accord with an expected Orbach type spin flip process [22] , [27] , [28] that is not considered further here. At lower temperatures u ( T ) becomes accurately proportional to 1/ T , which is consistent with the Nernst–Einstein equation for the Brownian diffusion of magnetic monopoles: Here, our transformed data indicates that the diffusion constant D is temperature-independent, as shown in the inset of Fig. 3d . The athermal diffusion constant shows that the observed temperature dependence of the magnetic relaxation [22] , in this temperature range, is completely accounted for by the temperature evolution of the monopole density, the isothermal susceptibility and the temperature factor characteristic of Brownian diffusion. This general behaviour is insensitive to small applied field (typically μ 0 H <50 mT, Fig. 3d ). Writing D = ν 0 a 2 /6 where a is the diamond lattice constant and v 0 the monopole hop rate [26] , [32] , we find a temperature-independent hop rate of ν 0 =2.43(6) × 10 3 s −1 . This athermal hop rate may be treated as evidence of quantum tunnelling of the spin involved in the monopole hop ( Fig. 1c ). Note that, owing to the several non trivial temperature-dependent terms in the expression for τ ( T ), it could be quite misleading to plot log( τ ) versus 1/ T ( Supplementary Fig. S2 ) as is commonly done when considering thermally activated relaxation processes: however, a treatment of this sort is given in Supplementary Note 3 . Our results are fully consistent with the theory of Ryzhkin [6] and the numerical analysis of Jaubert and Holdsworth [20] , which assumed an athermal hop rate, but also indicate an essential refinement that must be made to both these approaches. That is, we find a finite α , suggesting a significant dispersion of relaxation times, as previously observed [23] , rather than the single relaxation time assumed in the theory. However, the theory neglects monopole interactions (except insofar as they determine x ( T )), which might be expected to influence the hopping rate of individual monopoles. A detailed theory of such effects is far beyond the scope of this contribution, but we may derive a working model using the results of Bramwell [32] , where it was found that the mean square monopole field at a point is proportional to the monopole density. A heuristic argument for this is that the squared Coulomb field per monopole scales as 1/ r 4 (where r is distance) while the number of monopoles scales as xr 2 dr ; hence, neglecting monopole correlations, the mean square field scales as x times a finite definite integral over r . We assume that in zero applied field, spins are flipped by transverse fields [36] arising from the dense ensemble of atomic dipoles, and we decompose the instantaneous local transverse dipolar field as follows: where H 0 is an effective field that causes flipping at rate ν 0 . Here, h i ( i =1,2) are assumed to be uncorrelated random variables with zero mean and variance . Assuming τ −1 H , it follows that , for small h 1 , h 2 . Then using the additivity property of cumulants (here the variance) of uncorrelated random variables, we find Our measured α ( T ) may be transformed [37] to give the quantity on the left (Methods) and hence we can test the above expression. 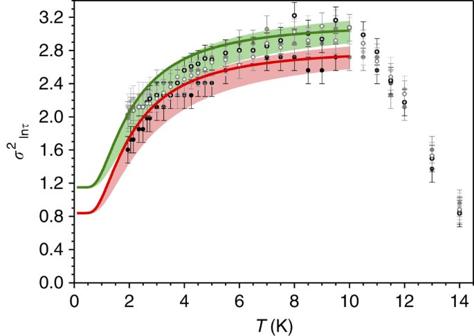Figure 4: Monopole signatures. The experimental variance in logarithmic relaxation time(circles, errors bars represent s.d.) compared with the predicted form for monopolar-field assisted tunnelling. Red and green indicate, respectively, applied fields ofand the set of finite fields listed in the caption ofFigure 3. For each curve there are two fitted parametersand, which describe the mean square static field and mean square monopole field, respectively. The line is the functionwherex(T) is the monopole density. The shading indicates the maximum possible systematic error (absolute minima and maxima) in the monopole density. We find σ1,2=0.84(1),3.40(5), respectively, in zero field and 1.15(1),3.40(5) in finite field. The deviation atT>10 K is related to a change in relaxation mechanism (see text). Figure 4 confirms a very satisfactory agreement between theory and experiment in zero and weak applied field, with the fitted σ 2 increasing rapidly in an applied dc field of 1mT, but thereafter more slowly. We may firmly conclude that the observed dispersion of rates is in large part a monopole property that obeys Equation 5. Given our derivation of Equation 5, our result suggests that monopole hopping is assisted by mutual monopole interactions, an inference that we examine further in the Supplementary Note 4 and Supplementary Fig. S3 . Figure 4: Monopole signatures. The experimental variance in logarithmic relaxation time (circles, errors bars represent s.d.) compared with the predicted form for monopolar-field assisted tunnelling. Red and green indicate, respectively, applied fields of and the set of finite fields listed in the caption of Figure 3 . For each curve there are two fitted parameters and , which describe the mean square static field and mean square monopole field, respectively. The line is the function where x ( T ) is the monopole density. The shading indicates the maximum possible systematic error (absolute minima and maxima) in the monopole density. We find σ 1,2 =0.84(1),3.40(5), respectively, in zero field and 1.15(1),3.40(5) in finite field. The deviation at T >10 K is related to a change in relaxation mechanism (see text). Full size image Isothermal and adiabatic susceptibilities The isothermal susceptibility χ T extracted from the fits to theory is in close agreement with the directly measured χ T ( Supplementary Fig. S4 ). At low temperature the isothermal susceptibility is predicted to be twice the Curie susceptibility [6] , χ T =2 C / T , but recent work [38] has established that in spin ice there is a gradual crossover from a Curie constant C at very high temperature to the expected 2 C at low temperature. Our results are consistent with a gradual evolution from χ T ≈1.8 C / T at T =2 K to χ T ≈1.2 C / T at T =10 K, consistent with this crossover, assuming a Curie constant of 3.95 K ( Supplementary Note 5 ). However a much more detailed experimental and theoretical study of the Curie Law crossover in Dy 2 Ti 2 O 7 would be worthwhile. The Curie like χ T is of course characteristic of a spin system: indeed there is no direct monopole signature in this quantity. This may be traced to the configurational entropy in the problem, which in applied field confines the monopoles [6] , [32] , making the magnetic response spin-like at long time. The thermodynamic adiabatic susceptibility χ S is the ac-susceptibility extrapolated to infinite frequency (or more strictly to a frequency where spin-spin relaxation is active but where spin-lattice relaxation is not [33] ). 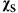Figure 5: Monopole and dipole signatures revealed by comparing the measured adiabatic () and isothermal () susceptibilities. (a) the susceptibilities are shown as a function of applied dc field at zero field (black circles) and near the crossover field (grey circles) shown as a red dotted line inFig. 1. Error bars represent s.d. The full red line is the experimentally measured monopole density fitted toby the adjustment of a scale factor (see text). The blue line is a Curie–Weiss law fitted to(Supplementary Fig. S4). The light blue line is the theoretical prediction(see text). (b) Measuredas a function of weak applied field(circles, same colour code is maintained as inFig. 3). The full red line is the experimentally measured monopole density fitted toby the adjustment of a scale factor (see text), also showing the maximum systematic uncertainty (absolute minima maxima) in the measured monopole density (red shading). Figure 5b illustrates a striking correlation between our measured adiabatic susceptibility χ S ( T ) and the measured monopole density x ( T ) (detailed checks on this result are given in Supplementary Note 6 and Supplementary Figs S5, S6 ). Thus, we find χ S = χ 0 x ( T ) with χ 0 =0.030(1), a temperature-independent constant. The athermal prefactor suggests that monopole diffusion is not involved in this magnetization process. Instead, in a simple classical interpretation, we may imagine a frictionless, and hence reversible, displacement of magnetic monopoles by distance r in the applied field—like a driven plasma oscillation. We write the force on a positive monopole as μ 0 H (ω) Q = Kr (ω), where K is the force constant, and use the fact that the magnetization is the magnetic moment per unit volume, or M (ω)=( x / V 0 ) Qr (ω). From these relations we find χ S = xμ 0 Q 2 / KV 0 , which is of the observed form, χ S x . From the value of χ S , we find K ≈0.06 N m −1 , implying an energy barrier between lattice sites at a distance r = a /2 of order 100 K. The latter seems too large to be a Coulombic barrier, and is more likely connected with the crystal field energy scale of several hundred kelvin. The amplitude of motion implied in our field of μ 0 H =5 × 10 −5 T is of the order of femtometres, which is much less than one lattice spacing. This frictionless oscillation of the monopole ensemble is reminiscent of a plasma oscillation in an electrical plasma, though the absence of an accelerative term in the equation of motion means that the monopole plasma oscillation cannot occur in the absence of a driving field. Of course a finite χ S in a magnetic system can always be formally represented as an oscillation of magnetic charge, but in this case the proportionality of χ S with x shows that it is associated with the displacement of recognizable positive and negative magnetic monopoles. Figure 5: Monopole and dipole signatures revealed by comparing the measured adiabatic ( ) and isothermal ( ) susceptibilities. ( a ) the susceptibilities are shown as a function of applied dc field at zero field (black circles) and near the crossover field (grey circles) shown as a red dotted line in Fig. 1 . Error bars represent s.d. The full red line is the experimentally measured monopole density fitted to by the adjustment of a scale factor (see text). The blue line is a Curie–Weiss law fitted to ( Supplementary Fig. S4 ). The light blue line is the theoretical prediction (see text). ( b ) Measured as a function of weak applied field (circles, same colour code is maintained as in Fig. 3 ). The full red line is the experimentally measured monopole density fitted to by the adjustment of a scale factor (see text), also showing the maximum systematic uncertainty (absolute minima maxima) in the measured monopole density (red shading). Full size image In a magnetic system χ S is always less than the isothermal susceptibility χ T , as it obeys the thermodynamic relation: where C H ≥0 is the specific heat at fixed applied field H . For an ideally paramagnetic rare earth salt a typical behaviour of χ S would be to roughly track the increase of χ T as T →0 according to the Curie Law χ T = C / T . The striking difference we observe between χ T ( T ) and χ S ( T ) ( Fig. 5a ) reflects a transition from spins to monopoles as the natural variables by which to describe the magnetic response, monopoles being more appropriate at high frequency. Nevertheless, we can explore the origin of χ S in spin language if we consider a monopole as a label for a set of ‘flippable’ spins ( Fig. 1 ). We assume that the adiabatic susceptibility is equal to the isolated susceptibility, which in a semi-classical approximation is given by [39] : Here, Z is the partition function, n labels the energy states of the system, and M n is the magnetic moment per unit volume of the state n . Our experimental observation that χ S = χ 0 x ( T ) is obtained if the ground state is assigned null adiabatic susceptibility and the monopole excited state is assigned ∂ M n /∂ H = χ 0 , where χ 0 is temperature independent. As M n = V −1 ∂ E n /∂( μ 0 H ) (where V is volume) our result reveals a quadratic term in the energy per monopole: . A quadratic energy expression generally indicates ‘stretchable’ magnetic moments. A small quadratic (Van Vleck) term is expected for a free Dy 3+ ion through mixing of the ground state with states of higher total angular momentum J . However, in our case, the observation that only flippable spins contribute to χ 0 and that flippable spins and non-flippable ones are distinguished only by a thermal energy scale at these temperatures, appears to rule out any single spin mechanism. It is interesting to note that the monopole spin texture is predicted to produce an electric dipole [40] and it appears from our result that it is associated with a magnetic polarizability as well. These findings have very important ramifications for the monopole description of spin ice. Previous work by neutron spin echo [27] , [28] on Ho 2 Ti 2 O 7 and μ SR (ref. 41 ) on Dy 2 Ti 2 O 7 has suggested a high frequency response that thermally evolves to low temperature, and that at first sight seems disconnected from the monopole picture. However, our results indicate that the dynamical spectrum in the approach to the high frequency limit is fully accounted for by magnetic monopoles, and they clearly explain the thermal evolution observed in the previous work. A very recent thermal conductivity study [42] indirectly estimates a diffusion constant for magnetic monopoles that is much faster than ours, but our adiabatic susceptibility results show that there is no necessary contradiction, as monopoles mediate a dynamical response over a very broad frequency range. Finally, our results rule out any significant spectral weight beyond that associated with monopoles, contrary to a recent proposal [43] . Adiabatic susceptibility in applied field Figure 1 shows the spin ice phase diagram for a dc-magnetic field applied along the cubic [111] direction. A small applied field orders one spin per tetrahedron in the pyrochlore structure, but maintains the ice rule of two spins in and two out per tetrahedron, thus creating the so called ‘kagome ice’ phase of two-dimensional disordered sheets, which still possess residual entropy [29] , [44] , [45] . With increasing field at T =0 there is a breaking of the ice rules, pictured as the flipping of one spin per tetrahedron, to create an ordered ‘three in, one out’ state. Extending from this point there is a line of first order phase transitions that terminates in a critical end point. The positive slope of this line reflects the destruction of the spin ice entropy by the applied field, according to the Clapeyron equation. In the monopole representation, the applied field tunes the chemical potential of monopole-antimonopole pairs such that the increased monopole density drives a first order condensation from a sparse monopole fluid to a dense ‘liquid’ (or perhaps better, ionic crystal) of alternating positive and negative monopoles [5] . The detailed theory of magnetic relaxation near the critical point [30] predicts mean field critical exponents modified by logarithmic corrections. Here, we are interested in the supercritical region at temperatures well above the critical point, where the system may be described as a dense monopole plasma. Recently, a peak in the ac-susceptibility at finite frequency was observed in this region [46] . We examined the behaviour of the adiabatic susceptibility as a function of field in this regime, to compare it with our zero-field measurement. In weak fields ( T) the thermal evolution of χ S ( T ) shows a slow increase with field, including a noticeable peak at higher temperature ( Fig. 6 ). In much stronger fields ( T) the adiabatic response is completely suppressed as would be expected ( Fig. 6 ), but at an intermediate field ( μ 0 H ≈0.920(8) T), χ S ( H ) exhibits a striking peak very near to the (internal) field of the zero temperature phase transition. At this field the ice rule is locally broken [44] and 1/4 of the spins in the sample may then be flipped at zero energy cost. However, in contrast to the zero-field result, χ S ( T ) measured near this crossover field (0.86 T) exhibits a simple Curie law, χ S = C ′/ T ( Fig. 5a ), indicating a different type of magnetic current to that observed in the weak field limit, as anticipated in Shtyk and Feigel’man [30] . We may regard the magnetic response in this regime as characteristic of switching magnetic dipoles, rather than magnetic monopoles. Note that the temperature evolution was measured at this point just off the peak maximum as it was found that systematic errors in fitting to the Cole–Cole function are minimized at this point ( Supplementary Note 6 ). The Curie constant C ′ may be calculated under the assumption that 1/4 of the spins are thermally active and that these have a projection of 1/3 of their full classical value on the field direction. Thus, we predict C ′= C /36=0.1097 where C ≈3.95 is the high temperature Curie constant. A fit of the experimental data to the expression χ S ( μ 0 H =0.86 T)= a /( T − T C ) gave a =0.090(5), T C =0.4(2) in close agreement with our prediction ( Fig. 5a ). 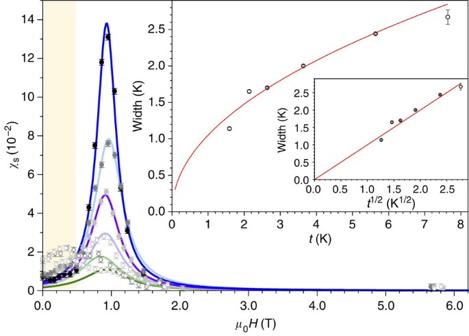Figure 6: Evidence of unconventional critical behaviour. Adiabatic susceptibility versus applied magnetic field, showing an unusual Lorentzian field dependence, suggestive of anomalous critical behaviour. The figure illustrates zero response at strong field and a peak at the field where the ice rule breaks. Error bars represent s.d. The lines are fits to a Lorentzian function at the following temperatures: blue,T=1.95 K; light blue,T=2.5 K; purple,T=3.0; lilac,T=4.0; light green,T=6.0; green,T=8.0 K. Scaling of Lorentzian width (Δ) (inset): the red line is the function. Experimental data appear to rule out the possibility of a different scaling—for example, linear scaleh/t. Figure 6: Evidence of unconventional critical behaviour. Adiabatic susceptibility versus applied magnetic field, showing an unusual Lorentzian field dependence, suggestive of anomalous critical behaviour. The figure illustrates zero response at strong field and a peak at the field where the ice rule breaks. Error bars represent s.d. The lines are fits to a Lorentzian function at the following temperatures: blue, T =1.95 K; light blue, T =2.5 K; purple, T =3.0 ; lilac, T =4.0 ; light green, T =6.0 ; green, T =8.0 K. Scaling of Lorentzian width (Δ) (inset): the red line is the function . Experimental data appear to rule out the possibility of a different scaling—for example, linear scale h / t . Full size image The striking 1/ T divergence and location of the peak position in the H−T plane ( Fig. 6 ) suggests that the adiabatic susceptibility is dominated by the classical critical point for monopole condensation ( Fig. 1 ), for which the isothermal susceptibility χ T is predicted [30] to diverge as 1/| T − T C | γ , with γ =1 and here. Usually the ratio χ T / χ S , analogous to the Landau–Placzek ratio in a fluid, should diverge towards the critical point. However, our data for χ T and χ S ( Fig. 5a ) illustrate a fairly typical paramagnetic response, as discussed above, with . Hence, both χ S and χ T diverge, but the latter is always larger, as required by thermodynamics (Equation 6). According to Shtyk and Feigel’man [30] , the field dependence of the susceptibility should be mean field like, with logarithmic corrections: hence, we would expect with δ =3. However, we observe an exponent of 2 rather than 2/3 ( Supplementary Fig. S7 ). Thus, defining reduced variables t = T − T C (with T C =0.36 K here), and h = H − H C , we find to a good approximation (suppressing dimensional constants): This implies scaling ( Fig. 6 , inset), which is formally characteristic of a zero dimensional phase transition ( Supplementary Note 7 ). An alternative interpretation of the field dependence is in terms of a classical single spin flip process, associated with the ‘free’ moments in the eventual ordered structure, which would be characterized by a response of the type and hence h/t scaling, but our data appear to distinctly rule against this possibility ( Fig. 6 , inset). Thus, the behaviour of χ S ( H ) seems inconsistent with both the ‘monopole’ and T =∞ fixed points. One possibility, as discussed further in Supplementary Note 7 , is that the susceptibility is dominated by a zero temperature quantum critical point, but again with anomalous exponents. It is noteworthy several other examples of anomalous exponents have been reported for the quantum critical behaviour of rare earth magnets [47] , [48] . Although the concept of magnetic monopoles in spin ice is supported by much experimental evidence [49] , [50] , [51] , the microscopic mechanism of monopole motion has yet to be identified. Our investigation of Dy 2 Ti 2 O 7 has isolated the characteristics of this mechanism to which any future theory must conform. Our first result is that, over the temperature ranged probed, monopoles obey the Nernst–Einstein equation with temperature independent diffusion constant, a strong signature of Brownian diffusion. It should be emphasized that this is an experimental result and not a theoretical input. We envisage Brownian diffusion in the sense of an electrolyte, where the motion of oppositely charged ions is strongly correlated, yet the Nernst–Einstein equation is obeyed if the Debye length is sufficiently small (as it is here) [32] . It would be useful to apply our methods to investigate monopole diffusion in the low temperature regime, as zero-field measurements in that regime await an unambiguous interpretation in the monopole picture [24] , [25] , and the theory of Shtyk and Feigel’man [30] has yet to be comprehensively tested. In this context we emphasize that the characteristic relaxation time τ ( T ) depends on at least three temperature-dependent factors, which shows that it cannot be treated in terms of an effective activation energy. However, our method disentangles all three factors and allows direct experimental estimation of the monopole mobility, which may be used to infer the monopole hop rate. We note a result [52] , [53] published while this paper was in final revision, that presents significant evidence of a low temperature (<1.5 K) crossover to a regime where the monopole hop rate is roughly proportional to monopole density (see also Castelnovo et al . [26] ). The precise temperature dependence of the hop rate can be experimentally determined by the general method presented here. It is interesting to discuss our result of Brownian motion in the context of band theory. Just as water ice can be thought of as an intrinsic protonic semiconductor [54] , so spin ice may be expected to be an intrinsic semiconductor for magnetic monopoles. These are produced by the thermal unbinding (or ‘fractionalisation’ [5] ) of conventional magnetic excitons. They tunnel from site to site and have an effective mass determined by the inverse Debye length (proportional [32] to ). However, one may ask the question, how are these expectations consistent with the diffusive motion of monopoles that our experiments have revealed? An answer might be found in the theory of Chen et al . [55] on the hopping of ionic defects in water ice, where it is shown how diffusive motion of defects can arise in a tight binding model that is constrained by the ice rules. Our second result is that the adiabatic susceptibility gives a clear perspective on the magnetic properties of spin ice, revealing a direct measure of the magnetic monopole concentration and critical behaviour in applied field. Our analysis of the adiabatic susceptibility has revealed a new property of magnetic monopoles: their partial magnetic polarization by an applied field. More generally we may conclude that the adiabatic susceptibility, often ignored as an uninteresting by-product of ac-susceptibility analysis, may contain a wealth of information about strongly correlated spin systems at low temperature. If we combine these results with the remarkable prediction that a monopole will carry an electric dipole moment (the equivalent of its spin, if we reverse the roles of electricity and magnetism) [40] a fascinating picture of the local properties of the monopole is starting to emerge. In general, the properties that we have discovered will have an important influence on any future application of magnetic monopoles in spin ice that seek to exploit their magnetic and thermal response. The dynamical magnetization of a 0.0326(1) g cubic crystal of Dy 2 Ti 2 O 7 was measured with the ACMS (AC-Measurement System) option of a PPMS (Physical Property Measurement System, Quantum Design). Alternating and dc magnetic fields ( H a c and H d c , respectively) were applied parallel to the cubic [111] axis of the sample. Data were collected at different temperatures between 1.9 K ≤ T ≤14 K in the ac-frequency range of 10 H z to 10 kHz. A variable dc field of μ 0 H =0−10 T was applied (at low field the absolute field was calibrated in dc-sweep measurement). Scans were taken at different ac fields in the range μ 0 H a c =0.05−3 × 10 −4 T to dispel the possibility of non-linear response of the system. The results presented here were taken at μ 0 H a c =5 × 10 −5 T. Data were corrected taking into account a demagnetizing factor to give . The calibrated response function of the instrument was checked by measurement of a very dilute paramagnetic salt ( Supplementary Fig. S5 , panel b and c). The data were fitted to the phenomenological model for the frequency dependent susceptibility described in (refs. 33 , 35 ). By separating Equation 2 it is possible to derive analytical expressions for the real and imaginary parts and Argand diagram (Cole–Cole plot), which were each fitted to the experimental data at a given temperature using a single set of parameters , , , . The Cole–Cole formalism assumes a symmetric unimodal distribution of logarithmic relaxation times with mean . It can be shown that [37] : In the text we label simply as for ease of reading, although strictly τ is a fixed parameter at a given temperature. It should be noted that there is no general way to derive the true mean relaxation time from ac-susceptibility data: here we approximate it to the Cole–Cole parameter τ . The dimensionless monopole density was estimated by fitting experimental specific heat data to Debye–Hückel theory [26] , [34] . The specific heat was represented as the temperature derivative of the energy per diamond lattice site: where is the monopole chemical potential, is the Debye-Hückel correction, calculated self consistently with the dimensionless monopole density , and is a correction for double charge monopoles. The experimental specific heat data, taken between , were fitted by adjusting , with the best fit value . The theory is not exact in the temperature range of interest and Figs 4 , 5 report an approximate envelope of systematic error, found by extrapolating the theory between low and high temperature according to different schemes ( Supplementary Note 1 ). How to cite this article: Bovo, L. et al . Brownian motion and quantum dynamics of magnetic monopoles in spin ice. Nat. Commun. 4:1535 doi: 10.1038/ncomms2551 (2013).